Ancient diversification ofHyposmocomamoths in Hawaii Island biogeography is fundamental to understanding colonization, speciation and extinction. Remote volcanic archipelagoes represent ideal natural laboratories to study biogeography because they offer a discrete temporal and spatial context for colonization and speciation. The moth genus Hyposmocoma is one of very few lineages that diversified across the entire Hawaiian Archipelago, giving rise to over 400 species, including many restricted to the remote northwestern atolls and pinnacles, remnants of extinct volcanoes. Here, we report that Hyposmocoma is ~15 million years old, in contrast with previous studies of the Hawaiian biota, which have suggested that most lineages colonized the archipelago after the emergence of the current high islands (~5 Myr ago). We show that Hyposmocoma has dispersed from the remote Northwestern Hawaiian Islands to the current high islands more than 20 times. The ecological requirements of extant groups of Hyposmocoma provide insights into vanished ecosystems on islands that have long since eroded. One of the most intriguing challenges in biology is the development of a timescale and robust paradigm for the process of speciation. Volcanic islands represent ideal study systems since they are impermanent platforms for evolution; as soon as the building phase is complete, they subside back into the ocean, eroding slowly until they disappear beneath the waves. Because of this dynamic process, endemic species radiations on remote volcanic islands are unique models for understanding the chronology of diversification in the framework of an isolated geological setting [1] . The Hawaiian Archipelago is the most isolated island chain on Earth, and is renowned as a site for the study of biogeography and speciation, in large part due to its remarkable geological history. All of its islands formed over a volcanic hotspot in the central Pacific, but as the Pacific plate carries them to the northwest, they move away from the relatively stationary source of magma. Once cut off from the magma, the islands gradually subside back into the ocean, becoming ever smaller rocky islets, pinnacles and finally coral atolls over the course of tens of millions of years. Thus, the islands are ordered linearly by age ( Fig. 1 ) [2] . The established ages of the islands, in concert with recent molecular clock advances, facilitate increasingly accurate time estimates of past speciation events. They provide powerful tools for unravelling the evolutionary history and impacts of geology on insular species radiations [3] , [4] , [5] . While the relatively young current high islands range in age from 0.5 (island of Hawaii) to 4.7 Myr ago (island of Kauai), the oldest of the persisting Northwestern Hawaiian Islands (NWHI), Kure atoll, is estimated at 29.8 Myr ago [2] , [3] . These ancient islands, some of which in their prime, rivalled the current high islands in size and topographic diversity, greatly extend the temporal window theoretically available for insular evolution in the Hawaiian Archipelago [2] . 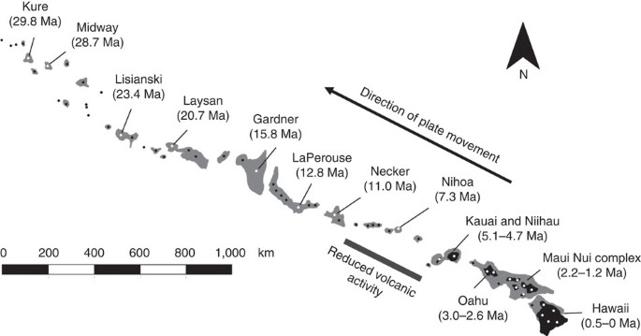Figure 1: Map of the Hawaiian Archipelago. Filled black areas represent current coastlines, while grey areas represent the maximum historical above-water island area. White dots correspond to volcanoes, peaks or small islands that are currently above sea level, while black dots indicate submerged seamounts. Note the lack of large islands between the islands of Necker (formed about 11.0 Myr ago) and Kauai and Niihau (formed 5.1–4.7 Myr ago). Figure reproduced with permission from the publisher, The Royal Society2. Figure 1: Map of the Hawaiian Archipelago. Filled black areas represent current coastlines, while grey areas represent the maximum historical above-water island area. White dots correspond to volcanoes, peaks or small islands that are currently above sea level, while black dots indicate submerged seamounts. Note the lack of large islands between the islands of Necker (formed about 11.0 Myr ago) and Kauai and Niihau (formed 5.1–4.7 Myr ago). Figure reproduced with permission from the publisher, The Royal Society [2] . Full size image However, the formation of the NWHI over the past 20 Myr ago was temporally inconsistent, which may have limited the survival and dispersal of ancient lineages [2] , [3] . By the time Kauai was formed ~5 Myr ago, it is thought that few (if any) of the older islands had peaks over 1,000 m in elevation [2] . It is assumed that low elevations severely limited precipitation on these islands, resulting in a much drier, less productive, archipelago that no longer supported diverse forest habitats or the organisms that depended on them. This theory depends partly on climatic patterns, which can vary considerably on the scale of thousands, let alone millions of years [6] . In addition to the lack of high mountains, there were two periods during which emerging islands were much more distantly spaced than at other times: 27–28 Myr ago and 5–7 Myr ago (just before the formation of Kauai, the oldest of the current high islands) ( Fig. 1 ). When Kauai formed, there were only relatively small, low islands available as sources, and the largest of these (Nihoa, Necker, LaPerouse and Gardner) were relatively distant compared with the spacing of the present high islands [2] . Thus, it is thought that distance and limited habitat variability on the source islands caused a ‘bottleneck’ that resulted in severe attrition in ancient lineages. Evidence from molecular clock studies generally supports this claim; Price and Clague [2] reviewed phylogenetic studies of Hawaiian plant and animal lineages, and found that the vast majority of age estimates were younger than the age of Kauai. This suggests that most endemic lineages that formerly occurred on the oldest islands did not persist, and diminishes the role that these atolls and pinnacles played in generating the archipelago’s present diversity, despite their greater size in the distant past. Only four extant lineages of plants or animals [7] , [8] , [9] , [10] are thought to have colonized the Hawaiian archipelago before the emergence of Kauai, but since all the living species in these apparently ancient lineages are currently restricted to the youngest islands, prior residence in the Hawaiian chain can only be inferred based on divergence time estimates. Moreover, very few of today’s species radiations have extant representatives on the NWHI, implying widespread extinction of ancient groups that never reached the younger islands, and thus extensive lineage turnover between islands greater than and those less than 5 Myr old. Understanding patterns of diversification in an ancient lineage would provide a unique perspective on the influence of time on island biogeography. The endemic Hawaiian moth genus Hyposmocoma is one of very few groups that maintain multiple single-island endemic species across the entire archipelago, including the NWHI. As such, this genus provides an unparalleled opportunity to examine the evolutionary history and island biogeography of an old, endemic radiation. Of particular interest, a group like Hyposmocoma offers a chance to include the role of the dwindling, ancient islands, many of which maintain their own endemic species. Hyposmocoma is a monophyletic radiation containing over 400 estimated species and accounting for one third of all butterfly and moth diversity in the Hawaiian Islands [11] . It represents one of the most spectacular and species-rich endemic radiations in the archipelago, second in numbers only to the Hawaiian Drosophilidae, which are largely restricted to relatively mesic habitats in the current high islands [12] . In contrast, Hyposmocoma occur on virtually every emergent landmass in the archipelago, and each species appears to be endemic to a single island. The moths have diversified into a wide range of habitats, from xeric lava fields along the ocean to high elevation bogs, fostering many novel adaptations, including unique amphibious [13] and carnivorous [14] case-making caterpillars. While many species of Hyposmocoma appear to be scavengers, they are specialized for different habitats, and this ecological diversity is reflected in the vast range of cases carried by the caterpillars [11] , although the selection pressures driving the diversity of cases are still unclear. The recent discovery of species belonging to several different lineages in the remote NWHI [15] , [16] suggests that the ancestors of the Hyposmocoma radiation may have colonized the archipelago long before the emergence of the main islands. An ancient colonization of Hawaii could partially explain the accumulation of such remarkable diversity, and would give insight into the importance of time in the generation of diversity. Further, by dating the divergence times for ecologically specialized species groups, it is possible to infer what ecological conditions existed on ancient source islands, which have long since eroded. Here we investigate the evolutionary history of this group, and its colonization patterns across the archipelago, using a systematic framework and molecular clock estimates from five genes, calibrated based on the geological history of the Hawaiian Islands. We report that Hyposmocoma is an ancient lineage, having diversified in the NWHI, and dispersed more than 20 times to the current high islands. Phylogenetic relationships The molecular phylogeny of Hyposmocoma recovers strongly supported species groups that, for the most part, correspond to nine distinct case types included in our analysis ( Fig. 2 ). The phylogeny supports the division of the genus Hyposmocoma into two previously recognized subgenera: Euperissus , whose larvae do not build cases, and Hyposmocoma sensu stricto, whose larvae build elaborate cases [11] . The basal lineages of Hyposmocoma sensu stricto have caterpillars that build cases with two entrances, one on each side, while a derived monophyletic radiation possess larval cases with a single entrance ( Fig. 2 ). 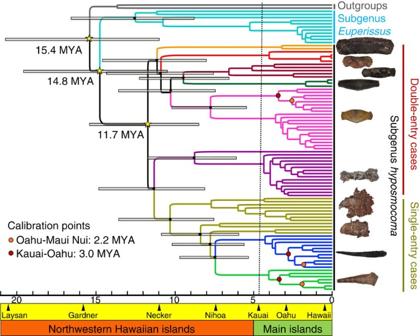Figure 2: Maximum clade credibility chronogram inferred using BEAST. The data set was combined for a total of 3,993 base pairs from five genes. BEAST was run for four replicates of 100 million generations, with sampling every 10,000 generations and discarding 50 million generations from each run as burn-in (total of 20,000 samples). The nine major case-type lineages are indicated by different colours, and calibration nodes are indicated by orange or red dots. Error bars represent 95% posterior credibility intervals and divergence times for major splits within the genus are indicated by stars. Ages are given in millions of years before present, with the emergence date of various islands indicated along the axis. Note that at the time of formation of Kauai (ca. 4.7 Myr ago), 24 of the extant lineages ofHyposmocomahad already split, and all of these now occur in the high islands, implying 24 independent dispersal events from the NWHI to the current high islands. Figure 2: Maximum clade credibility chronogram inferred using BEAST. The data set was combined for a total of 3,993 base pairs from five genes. BEAST was run for four replicates of 100 million generations, with sampling every 10,000 generations and discarding 50 million generations from each run as burn-in (total of 20,000 samples). The nine major case-type lineages are indicated by different colours, and calibration nodes are indicated by orange or red dots. Error bars represent 95% posterior credibility intervals and divergence times for major splits within the genus are indicated by stars. Ages are given in millions of years before present, with the emergence date of various islands indicated along the axis. Note that at the time of formation of Kauai (ca. 4.7 Myr ago), 24 of the extant lineages of Hyposmocoma had already split, and all of these now occur in the high islands, implying 24 independent dispersal events from the NWHI to the current high islands. Full size image Divergence time estimates The relaxed molecular clock analysis estimates the basal divergence within the monophyletic genus Hyposmocoma at 14.8 Myr ago (10.5–19.6, 95% highest posterior density (HPD)) ( Fig. 2 ), establishing its arrival time well before the formation of the current high islands. While the date of the original colonization could be older, this represents the earliest divergence among extant Hyposmocoma species, making this a conservative estimate of the age of the lineage, and one of the oldest ages estimated for a Hawaiian lineage using modern calibration methods. The analysis estimated the divergence between Hyposmocoma and the cosmopterigid genera Labdia and Limnaecia at 15.4 Myr ago (11.0–20.7, 95% HPD), giving an upper limit for the date of colonization. Taking into account the error associated with these two estimates, the analyses suggest that colonization occurred between 10.5 and 20.7 Myr ago. Further, the phylogeny implies that splits among all nine of the basic Hyposmocoma case types occurred prior to the emergence of any of the current high islands, and many of these case types dispersed to the high islands multiple times. In sum, our results suggest that at least 24 independent colonists from the genus Hyposmocoma dispersed from the NWHI to the current high islands, and their descendants persist to the present day. The geological window for initial colonization and diversification within the group corresponds to the first ‘peak period’ in the archipelago (8.0–18.0 Myr ago), when multiple, now-vanished volcanoes were more than 1,000 m above sea level [2] . A colonization around 14.8 Myr ago would have occurred soon after the formation of Gardner Pinnacles (15.8 Myr ago), which was the largest of the now-submerged volcanoes in the NWHI, exceeding 4,000 m elevation at its peak size, and comparable in land area with the current largest island of Hawaii [2] . The basal position of extant NWHI species within lineages offers additional strong evidence that major case-type lineages arose within the NWHI, and are not the result of back-colonization. In particular, the ‘cone’ clade includes species from Laysan, Necker and Nihoa [16] , and all three of these are recovered as basal branches to the rest of the clade. This is not only true in the tree produced by the concatenated data set ( Supplementary Figs 1 and 2 ), but also in trees constructed using data from each of the five individual genes ( Supplementary Figs 3–7 ). Substitution rates Rates of divergence for each partition are shown in Supplementary Table 1 . As expected for protein-coding genes, mean substitution rates were highest for third codon positions and lowest for second codon positions in both mitochondrial and nuclear genes. For the mitochondrial gene CO1, which has been widely used in molecular clock estimations, our calibrations resulted in a mean rate of 8.8% pairwise divergence per Myr. This rate is nearly four times higher than the commonly used ‘standard’ rate of evolution for CO1 in insects, 2.3% per Myr [17] . Generally, divergence rates for CO1 fall within the range of 0.5–4% per Myr [18] , although Roesch Goodman et al . [19] compiled a wider range of rates (1.3–10.6% per Myr) for divergences between sister species in a diversity of Hawaiian arthropod groups. Our high mean rate of evolution in CO1 compared with other studies either implies a faster rate of mutation in CO1 in Hyposmocoma or suggests that our age estimates are underestimates. If we were to apply the ‘standard’ rate of 2.3% per Myr, the resulting age estimate for Hyposmocoma would be substantially older, consistent with our conclusion that it is an ancient lineage. However, given the documented high variability of rates of evolution across invertebrate taxa [20] , we feel that the application of a so-called ‘standard’ rate is somewhat arbitrary, although it can provide useful rough estimates when calibrations are not available. Divergence rates for the pooled nuclear data set were considerably lower than for CO1 ( Supplementary Table 1 ), with a mean rate of 0.6% pairwise divergence per Myr. Most of the genes we used have not been widely used for divergence time estimations, and there are therefore no accepted ‘standard’ rates for these genes. The basal diversifications in Hyposmocoma long predate the bottleneck in island formation that ended with Kauai 4.7 Myr ago; at that time, there were no large islands and the largest remaining island, Gardner Pinnacles, was over 1,000 km from Kauai, and had eroded to less than 1,500 m elevation. Thus, our results imply that over twenty Hyposmocoma colonists dispersed from a small island (or multiple small islands) across this gap, which is thought to have been insurmountable for most other NWHI flora and fauna [2] . Considering that this gap in island formation acted as a dispersal filter, the extant lineages of Hyposmocoma likely represent a subset of the case types that existed in the NWHI. All of the NWHI are now severely eroded, a few marked by atolls, suggesting that Hyposmocoma lineages derived on those once high islands were some of the few organisms that migrated down the island chain, tracking the rising, younger, higher islands in an unbroken succession of dispersals over millions of years. While the vast majority of extant Hyposmocoma species are the result of relatively recent diversification after the young, high islands arose, the nine basic case-type lineages all evolved well before the newest islands ( Fig. 2 ), suggesting that much of the ecological diversity of Hyposmocoma evolved very early on. In contrast, more recent diversification within the high islands appears to be largely driven by the process of dispersal to, and subsequent isolation on, new islands, as opposed to purely being driven by niche partitioning. This is evidenced by ecological conservation within but not across lineages within the genus (for example, carnivorous caterpillars are monophyletic and their inception predates the current high islands). The varying ecological specialization of Hyposmocoma on a lineage level provides indirect evidence for the environmental conditions and a reflection of habitats available on past high islands, and, by extension, similarity to those on the current high islands. This is a strong evidence for the profound evolutionary significance of volcanoes now vanished beneath the Pacific Ocean, and the contribution of past island biogeography to the current biota. The chronology and patterns of diversification driven by now-obscured geological history likely play a fundamental role in the current biogeographic patterns in other groups, both insular and continental. For the most part, the Hyposmocoma lineages that currently survive on the bleak NWHI represent basal branches within lichen-grazing, rock-inhabiting groups. Most forest-dwelling species groups (for example, tree snail-eating caterpillars and rotting-wood borers, comprising more than 60 species) are no longer present, but molecular dating suggests that they all evolved in the NWHI ( Fig. 2 ). It is parsimonious to assume that these diverse forest-dependent lineages have long depended on forests for their survival, suggesting that the ancient atolls and pinnacles not only once supported forests, but that these habitats persisted until the formation of Kauai (about 5 Myr ago). Since a diverse assemblage of plant and animal lineages likely occurred on the NWHI, the reasons for their apparent failure to reach the younger islands, and the resulting massive turnover, not just in species, but in lineages, is unclear. This phenomenon is especially perplexing considering that Hyposmocoma has successfully colonized the current high islands over 20 times, and has persisted for millions of years. This suggests that either distance was not a critical factor limiting the dispersal of other groups from the NWHI, or Hyposmocoma , despite being tiny micromoths, are unusually vagile. Island biogeography has focused on adaptive radiations [21] , [22] as a dominant mechanism generating new species. Under this model, a founder arriving on a new island radiates into a variety of species with distinct niches. Thus, a limited number of founders diversify into a variety of forms and habitats. At the least, this should manifest itself as the evolution of ecological diversity in rapidly speciating lineages [23] . It is clear that Hyposmocoma has undergone dramatic diversification into highly partitioned niches, as evidenced by the different case-type lineages that correspond to different feeding behaviours and habitats [13] , [14] , [15] . However, for the most part, this ecological diversification occurred long ago, with all major case types diverging prior to 7 Myr ago ( Fig. 2 ), suggesting that the major ‘adaptive’ part of this radiation happened early in the evolutionary history of this group. The degree to which diversification continues to be driven by or associated with ecological specialization is unclear. Hyposmocoma species are virtually all island endemics, and recent speciation appears to be precipitated primarily by colonization of new islands and regions, followed by geographic isolation. To some degree, ecological specialization no doubt continues to drive speciation, but perhaps not as strongly as it did following initial colonization of the islands. Hyposmocoma may not be an exception to the general pattern of recent colonization put forward by Price and Clague [2] , but rather one of the few groups for which an ancient evolutionary history can be recovered, due to a large number of dispersal events. Most age estimates for Hawaiian lineages are based on relationships among extant Hawaiian taxa, rather than comparisons with a sister taxon outside of Hawaii. As acknowledged by Price and Clague [2] , it is impossible to demonstrate an age older than Kauai for a given lineage unless at least two ancestors with extant descendants have dispersed from the NWHI to the current high islands. If a lineage was the product of a single dispersal event from the NWHI to Kauai, the resultant phylogeny would be indistinguishable from that produced by a colonization from outside Hawaii; in both scenarios, basal divergences among extant Hawaiian taxa would occur after the formation of Kauai. It is quite possible that the accepted ages of many Hawaiian lineages are underestimated, and many may be the result of a single dispersal event from the NWHI. The only way to definitively establish that a Hawaiian lineage is, in fact, younger than Kauai is if the divergence between it and a close external relative occurred less than 5 Myr ago. Unfortunately, for most lineages, this has not been shown, and identifying an appropriate extant sister taxon outside of Hawaii is not always straightforward or possible, especially in invertebrates, which are often diverse and little studied. This is not a criticism of other studies, but merely an acknowledgement of the limitations imposed by the available data. Hyposmocoma provides evidence that colonization from the NWHI not only occurred, but occurred repeatedly, suggesting that dispersal in other groups may have occurred more often than we can detect. The divergence time estimates reviewed by Price and Clague [2] were primarily for bird and plant lineages. Only two studies of insect lineages (drosophilid flies and damselflies) were cited, and both of these suggested colonization prior to the formation of Kauai [8] , [9] , although more recent studies have shown that some species-rich insect lineages are the product of very recent colonization [24] , [25] . The Hawaiian biota boasts extremely high endemism, not only on the species level, but on higher taxonomic levels as well. All major groups of organisms include endemic Hawaiian genera [10] , [11] , [26] , and the existence of so many endemic higher taxa implies long isolation from their continental relatives. Because Hyposmocoma represents a third of all Hawaiian lepidopteran diversity, and is one of the most diverse genera of any kind on any volcanic archipelago, its pattern of diversification is broadly relevant to island biodiversity. While Hyposmocoma represents a small fraction of lineages that became hyperdiverse, such lineages now constitute the majority of overall species diversity. The success of Hyposmocoma illustrates the importance of alternative diversification patterns, beyond adaptive radiation-driven speciation, in generating and maintaining insular biodiversity, and detailed investigation of more recent speciation patterns will shed light on how the processes fostering diversification within a group can change over time. Sampling All adults for this study were reared in the lab from case-making caterpillars to confirm ecological affiliations. Larvae were collected from across the islands of Hawaii, Kauai, Lanai, Maui, Molokai and Oahu, as well as on the older NWHI of Laysan, Necker and Nihoa. We reared each collection of Hyposmocoma larvae in Petri dishes and larvae were typically fed carrot and commercial TetraMin fish food. Some larvae with more specialized feeding habits were offered lichen, rotten wood or Drosophila pupae. For each field collection, a unique data log entry was made including date and location, digital pictures of larvae and case, record of larval behaviour, date of adult moth emergence and digital picture of adult moth. Adult moths were then frozen at −80 °C for molecular sequencing. Prior research confirms that Hyposmocoma is clearly monophyletic [13] . We sampled broadly across the lineages of Hyposmocoma , including 90 species out of ~350 described, including 79 species from subgenus Hyposmocoma, representing all case-type lineages, and 11 species from subgenus Euperissus , which do not construct cases. Because each lineage has multiple species, each endemic to a different island, we focused on the broadest ecological and morphological range of species in our sampling to make sure all lineages were represented. Naturally, extinction of lineages or poor sampling distribution might influence the estimates of age and relationship across the group, but assuming we captured most of the diversity, these estimates would most likely end up being underestimates of the true age of Hyposmocoma , rather than exaggerations. To root trees and estimate divergence times from non-Hawaiian relatives, we included cosmopterigine moths from two other genera: Labdia issikii and Limnaecia sp. Although the closest relatives for Hyposmocoma have not been established, and generic relationships within Cosmopterigidae worldwide have not been studied, Zimmerman [11] proposed these two genera as possible sister taxa to Hyposmocoma . Of the cosmopterigine taxa available to us, these were placed nearest to Hyposmocoma by preliminary analyses. Molecular sequencing Whole genomic DNA was extracted from the thorax, head or legs from adult moth specimens using the DNeasy blood and tissue kit (Qiagen). Bodies were conserved as vouchers and deposited in the University of Hawaii Insect Museum, Honolulu, USA). Detailed data on collection localities and DNA GenBank accession numbers ( KJ440092 to KJ440488 in the nucleotide database) of all sequences are listed in Supplementary Table 2 . Using polymerase chain reaction (PCR), fragments of five genes were amplified: the nuclear genes EF-1α, CAD, MDH and RpS5, and the mitochondrial gene CO1. 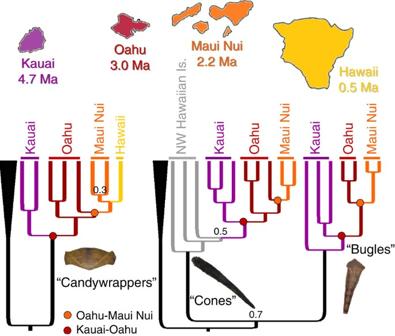Figure 3: Phylogenies of threeHyposmocomacase-type lineages used to calibrate divergence time analyses. Clades are excised from a larger, 90-taxa Bayesian tree obtained in BEAST without enforcing age calibrations, and unless otherwise indicated, posterior probability for nodes exceeds 0.98. The internal calibration points chosen for divergence time estimation represent inferred dispersal events from Kauai to Oahu (red dots) and from Oahu to Maui Nui (orange dots). The Maui Nui complex is composed of four islands (Kahoolawe, Lanai, Maui and Molokai) that were historically connected. Primers and their annealing temperatures are listed in Supplementary Table 3 . Thermal profiles for PCR started with 2 min of denaturation at 95 °C, followed by 35 cycles of denaturation at 95 °C for 1 min, an annealing step for 1 min and elongation at 72 °C for 1 min. Cycles were followed by a final step for 12 min at 72 °C. Amplified PCR products were purified using the QIAquick PCR Purification kit (Qiagen) and run on an ABI Prism 377 XL automated DNA sequencer. The final data set consisted of a total of 3,993 base pairs (bp), including CO1 (1,422 bp), EF1a (771 bp), CAD (705 bp), MDH (498 bp) and RpS5 (597 bp). Phylogenetic analyses Sequences were unambiguous and without insertions or deletions, and therefore easily assembled manually, edited and aligned with Geneious version 5.5.6 (ref. 27 ). We assessed whether sequence data from the five genes were compatible by running an Incongruence Length Difference [28] test in TNT v. 1.1 (ref. 29 ) with 1,000 replicates, which found no significant difference among data from the five genes ( P =1.0), justifying their concatenation into a single partitioned data set. As an additional qualitative assessment of the congruence among genes, we constructed trees for each gene using a maximum likelihood optimality criterion in the programme GARLI (Genetic Algorithm for Rapid Likelihood Inference) [30] v. 2.0 implemented using the GARLI web service [31] . For evaluation of gene trees, we performed unpartitioned analyses, due to the short length of individual gene sequences, and concerns about overpartitioning. For each tree, we ran 10 GARLI replicates to obtain the best tree, followed by 1,000 bootstrap replicates to assess support for tree topologies. Because we found no evidence of divergent evolutionary histories among genes ( Supplementary Figs 3–7 ), we combined all five genes into a single data set partitioned by organelle (mtDNA or nDNA) and codon position, for a total of six partitions. We selected the best model of evolution for each partition using the corrected Akaike information criterion computed in jModelTest [32] . Models selected were as follows: mt1, SYM+I+G; mt2, HKY+I; mt3, HKY; nuc1, GTR+I+G; nuc2, GTR+I+G; nuc 3, GTR+I+G. Phylogenetic analyses were performed using the programme BEAST v1.7.5 (ref. 33 ) and associated software (Beauti v1.7.5, Tracer v1.5, LogCombiner v1.7.5, TreeAnnotator v1.7.5) [33] for dating analyses in a Bayesian framework. BEAST analyses were run through the online CIPRES Science Gateway [34] . Analyses were run using a lognormal relaxed clock and the Yule model of speciation, and BEAST was set to estimate site and clock parameters independently and simultaneously with each gene partition. A run was also performed without data, to assess prior distributions and allow comparisons with posterior distributions. The Markov chain Monte Carlo in BEAST was run for 100 million generations and sampled every 10,000 generations. Four replicate runs were performed to check for convergence of the Markov chain Monte Carlo and combined together after discarding 50 million generations from each run as burn-in. The effective sample size of each parameter, viewed in Tracer, indicated the number of effectively independent iterations represented by each run and reflected how well the samples estimated the posterior distribution for each parameter. We assessed confidence in tree topologies as posterior probabilities calculated for each node. We also performed maximum likelihood analyses of the concatenated data set in GARLI, as described above, using the same partitioning scheme and model settings used for BEAST analyses. Molecular clock calibration Previous analyses showed that three clades distributed across the Hyposmocoma phylogeny showed strong evidence of the ‘progression rule’. In other words, evolution progressed in a stepwise fashion down the island chain, with taxa from older islands diverging basally, and taxa from younger islands diverging more recently. These clades were the ‘candywrapper’, ‘cone’ and ‘bugle’ cases, from which we included species endemic to each of the main Hawaiian Islands ( Fig. 3 ). We calibrated two nodes in each of these clades, which corresponded to presumed dispersal events from older islands to younger islands, for a total of six calibration points. The priors for these nodes were assigned a normal distribution with a relatively wide s.d., as recommended for calibrations based on geological ages [35] . This allows flexibility around calibration points, since actual divergence times among extant island taxa can either precede the formation of the younger island (if ancestral populations diverged prior to dispersal) or lag behind it (if dispersal does not occur soon after island formation). This approach assumes that dispersal from older islands to younger islands occurred soon after the formation of the new island, and therefore is only appropriate when calibration clades show overwhelming evidence of the progression rule. The six nodes chosen included three representing dispersal from Kauai to Oahu and three representing dispersal from Oahu to Maui Nui. Kauai–Oahu dispersal events were calibrated by setting the prior for that node to 3.0 Myr ago with a s.d. of 1.0, while Oahu–Maui Nui dispersals were calibrated at 2.2 Myr ago with a s.d. of 0.73. Calibrations were assigned generous standard deviations (1/3 island age) to allow for push and pull among the multiple calibrations, since actual divergences among extant taxa may have occurred either before or after island formation [35] . We elected not to include a seventh presumed dispersal event from the NWHI to Kauai in the ‘cone’ clade ( Fig. 3 ) as a calibration point in the analyses, to avoid circularity of conclusions about the role of the NWHI as a colonization source. Figure 3: Phylogenies of three Hyposmocoma case-type lineages used to calibrate divergence time analyses. Clades are excised from a larger, 90-taxa Bayesian tree obtained in BEAST without enforcing age calibrations, and unless otherwise indicated, posterior probability for nodes exceeds 0.98. The internal calibration points chosen for divergence time estimation represent inferred dispersal events from Kauai to Oahu (red dots) and from Oahu to Maui Nui (orange dots). The Maui Nui complex is composed of four islands (Kahoolawe, Lanai, Maui and Molokai) that were historically connected. Full size image Following analyses, posterior distributions of calibration nodes were compared against prior distributions to assess conflicts among calibration points. Ages of various nodes were estimated from the resulting tree, using the 95% HPD as an estimate of error for the age of each node. How to cite this article: Haines, W. P. et al . Ancient diversification of Hyposmocoma moths in Hawaii. Nat. Commun. 5:3502 doi: 10.1038/ncomms4502 (2014). Accession codes : Novel DNA sequences generated during this study have been deposited in the GenBank nucleotide database under the accession codes KJ440092 to KJ440488 .